Observation of a universal donor-dependent vibrational mode in graphene Electron–phonon coupling and the emergence of superconductivity in intercalated graphite have been studied extensively. Yet, phonon-mediated superconductivity has never been observed in the 2D equivalent of these materials, doped monolayer graphene. Here we perform angle-resolved photoemission spectroscopy to try to find an electron donor for graphene that is capable of inducing strong electron–phonon coupling and superconductivity. We examine the electron donor species Cs, Rb, K, Na, Li, Ca and for each we determine the full electronic band structure, the Eliashberg function and the superconducting critical temperature T c from the spectral function. An unexpected low-energy peak appears for all dopants with an energy and intensity that depend on the dopant atom. We show that this peak is the result of a dopant-related vibration. The low energy and high intensity of this peak are crucially important for achieving superconductivity, with Ca being the most promising candidate for realizing superconductivity in graphene. The fundamental interplay of electrons and phonons mediates superconductivity [1] in the conventional superconductors [2] and also plays an important role for many properties of undoped cuprates [3] . Angle-resolved photoemission (ARPES) has become an important tool that allows to probe electron–phonon coupling (EPC) as a kink in the spectral function of a material. The investigation of EPC in graphene [4] is promising due to graphene’s simple structure and the ease by which it can be functionalized chemically to tune its electronic properties [5] , [6] , [7] , [8] , [9] . If graphene is on a metal surface, electron–electron interaction is considerably reduced due to screening by the substrate [10] . Regarding EPC, superconductivity in graphene has not been reported experimentally yet, despite EPC induced superconductivity was found in many other carbon-related materials like intercalated graphite (GIC) [11] , fullerene crystals [12] , [13] , [14] , [15] , nanotubes [16] and boron-doped diamond [17] . In these systems, the common way to achieve superconductivity is electron doping that enlarges the Fermi surface and hence the phase space contributing to EPC, leading to an enhanced T c . For the graphene-derived GICs, the shape of the Fermi surface is crucially important: an incomplete ionization and hence a partially occupied dopant-derived electronic band is a key for getting high values of T c (ref. 18 ). The dopant-derived free-electron like band can efficiently couple to out-of-plane graphene phonons and in-plane dopant phonons and hence increase the total EPC [19] , [20] , [21] . The low energy of the phonons is particularly helpful for generating large coupling since the EPC is proportional to the inverse phonon energy. The physical reason behind this is the larger amplitude for low-energetic vibrations and hence a larger orbital overlap change. As for graphene, the condition regarding the interlayer band also holds but is modified due to the absence of a confining potential. Hence, the wavefunction of the interlayer state has a different shape. This can lead to marked increases in T c as theoretically predicted for Li-covered graphene [22] , which is expected to have T c =8.1 K. For intercalated bilayer graphene, the dopant/carbon stoichiometry is lower and new breathing-like phonons exist, where layers vibrate against each other. These have a substantial EPC to the interlayer state that can partially compensate for the lower doping. For example, the C 6 CaC 6 bilayer is predicted to superconduct with T c values approaching the ones of bulk CaC 6 (ref. 23 ). In summary, the above theoretical models for achieving high EPC in graphene rely on (i) large doping, that is, divalent alkaline earth metals are preferred, (ii) an ordered dopant which induces interlayer band formation and (iii) a suitable shape of the interlayer band wavefunction. Regarding (i) and (ii), previous results [24] , which are confirmed in our present work, state that Ca does not form an ordered phase when deposited onto monolayer graphene. However, an ordered phase of intercalated Ca atoms has been reported for bilayer graphene [25] . It therefore appears that the intercalation process is important for achieving dopant order. Regarding (iii), for quasi-free-standing graphene on a substrate, the location of the dopant with respect to the interface (on top of graphene or in the substrate/graphene interface) has a presumably large influence on the interlayer state’s wavefunction. In view of the above points, we direct our efforts towards the search of a system with large EPC, which can sustain superconductivity with graphene’s π bands alone. To that end we employ the ARPES technique to evaluate the electronic band structure and to extract the Eliashberg functions [26] , [27] of graphene doped with Cs, K, Na, Rb, Li and Ca. The results clearly show an emerging low-energy peak whose position depends on the dopant atom, indicating coupling to a dopant-derived vibration. In combination with the large charge transfer from Ca, its phonon makes a large contribution to EPC and can hence facilitate superconductivity at 1.5 K in Ca-doped graphene. Interface geometry Fully doped graphene samples were synthesized in situ as described in the Methods section. We investigate the position of the dopant atom (Cs, K, Rb, Na, Li, Ca) by angle-resolved x-ray photoelectron spectroscopy (XPS) measurements of the C 1 s and dopant core level spectra, which are highly sensitive to the element position in z direction ( z is perpendicular to the graphene layer). In Fig. 1 we show the dopant and carbon core level spectra probed in normal emission and grazing emission as it is displayed in the inset. This method allows to determine the carbon/metal stoichiometry and the location of the dopant atom (inside the Au/graphene interface or on top of graphene) via the relative photoemission intensities for normal and grazing emission [27] . From the ratios shown in Fig. 1 , it is clear that there is a qualitative difference between K, Ca and Cs, Rb, Na, Li dopants. For the former case of K and Ca, the signal in normal emission is stronger when compared with grazing emission while in the latter case this ratio is inverted. Hence, the current experiments conclusively show that only K and Ca intercalate into the graphene-Au interface, and Cs, Rb, Na and Li are preferably located on top of graphene. While the structure of the alkali metal core level spectrum is relatively simple and only changes in intensity when going from normal to grazing emission (see for example K 2 p ) the case of Ca is more complicated because Ca alloys with Au. The XPS of the Ca 2 p spin doublet reveals at least two different states, Ca s and Ca b for normal emission and one additional state, Ca c for grazing emission. The component Ca c is shifted to lower binding energy and almost absent in the case of normal emission, which points towards a high surface character such as due to small Ca clusters on top of graphene. The other components show a behaviour consistent with intercalated Ca and one can find that the intensity of Ca s decreases less than Ca b with respect to the emission angle. Hence, the behaviour of Ca s suggests that it corresponds to a Ca layer under the graphene sheet, while Ca b corresponds to Ca that forms an alloy with the Au substrate. 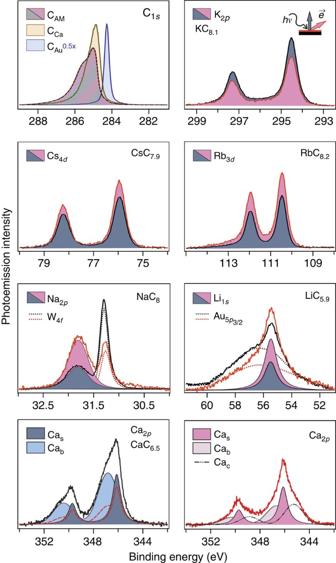Figure 1: Angle-dependent x-ray photoelectron spectroscopic characterization. Core-level spectra in normal and grazing emission geometry for each dopant and the corresponding graphene C1score-level spectra. The C1score-level spectra of graphene on Au (CAu), alkali-metal-doped graphene (CAM) and Ca-doped graphene (CCa) are shown. The inset to the upper right subfigure denotes the experimental geometry. For the normal emission spectrum of Ca2p(bottom left graph), the red, dashed lines indicate the Casand Cabpeaks of grazing emission. See text for details. The carbon/dopant stoichiometries determined by the XPS intensity ratios are indicated for each dopant. Figure 1: Angle-dependent x-ray photoelectron spectroscopic characterization. Core-level spectra in normal and grazing emission geometry for each dopant and the corresponding graphene C 1 s core-level spectra. The C 1 s core-level spectra of graphene on Au (C Au ), alkali-metal-doped graphene (C AM ) and Ca-doped graphene (C Ca ) are shown. The inset to the upper right subfigure denotes the experimental geometry. For the normal emission spectrum of Ca 2 p (bottom left graph), the red, dashed lines indicate the Ca s and Ca b peaks of grazing emission. See text for details. The carbon/dopant stoichiometries determined by the XPS intensity ratios are indicated for each dopant. Full size image We found that the graphene C 1 s core level spectra are strongly affected by the doping. We observe (i) a shift to higher binding energies by ∼ 0.8 eV for the alkali metals and by ∼ 0.6 eV for Ca and (ii) the C 1 s line changes shape. Regarding (i) the shift towards higher binding energies is smaller than the coresponding valence band shifts and is ascribed to core-hole screening. Regarding (ii) the change in lineshape upon doping is well known for carbon materials and is due to the coupling to conduction electrons, which induces the asymmetric Fano lineshape. The difference in the C 1 s line shapes for the alkali metals and Ca may be due to screening effects and chemical shifts in the alkali atoms due to their diverse environment, for example, Ca is partially alloyed with Au. Electronic structure To evaluate how much charge each dopant is able to transfer to graphene, we performed ARPES measurements of the Fermi surface and cuts in the energy-momentum space along the Γ KM high symmetry direction. To ensure that the samples investigated correspond to maximally doped graphene, we performed stepwise evaporation of dopants onto graphene followed by ARPES measurements of the Fermi surface. Only if the Fermi surface area did not increase upon doping, we considered the doping level reached to be the maximum. The ARPES data sets of fully doped graphene are presented for all dopants in Fig. 2a . The number of extra electrons per C atom is readily calculated from the ratio of the Fermi surface area to the area of the Brillouin zone and displayed inside each dopant’s Fermi surface. It is not surprising that the highest charge transfer occurs for Ca-doped graphene since Ca is able to offer its two valence electrons to graphene while all other dopants have only one. Let us now look to the modifications of the band structure that lie beyond the aforementioned doping effect. 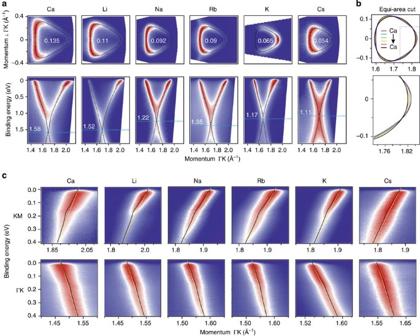Figure 2: The ARPES intensities of doped graphene. (a) ARPES spectra of maximally doped graphene for different dopants. The black dotted line denotes the ARPES intensity maxima. Upper row: Fermi surfaces and electrons transferred per C atom (values inside the contour). Data are acquired ins-polarization for Ca, Li, Na, Rb, Cs and inp-polarization for K doping. Lower row: ARPES scans along the ΓKMhigh symmetry direction in the vicinity ofKpoint (at 1.7 Å−1), summing the data forsandppolarization. The numbers give the energy of the Dirac points. (b) Iso-area contours for all dopants and magnification along theKMhigh symmetry direction. (c) High resolution ARPES data in the kink region forKMand ΓKdirections measured inp- ands-polarization, respectively. The yellow lines give the bare-particle band structure. Figure 2: The ARPES intensities of doped graphene. ( a ) ARPES spectra of maximally doped graphene for different dopants. The black dotted line denotes the ARPES intensity maxima. Upper row: Fermi surfaces and electrons transferred per C atom (values inside the contour). Data are acquired in s -polarization for Ca, Li, Na, Rb, Cs and in p -polarization for K doping. Lower row: ARPES scans along the Γ KM high symmetry direction in the vicinity of K point (at 1.7 Å −1 ), summing the data for s and p polarization. The numbers give the energy of the Dirac points. ( b ) Iso-area contours for all dopants and magnification along the KM high symmetry direction. ( c ) High resolution ARPES data in the kink region for KM and Γ K directions measured in p - and s -polarization, respectively. The yellow lines give the bare-particle band structure. Full size image Generally speaking, band structure modifications stem from (i) electron–phonon coupling, (ii) electron–plasmon coupling, (iii) electron–electron interactions and (iv) modifications of the underlying bare-band structure due to the presence of the positively charged ions. The renormalizations that occur from electron–phonon coupling are at ∼ 180 meV below the Fermi level and will be discussed in detail in the next section. The renormalizations due to electron–plasmon coupling are pinned to an energy close to the Dirac point [28] . Regarding electron–electron interactions, they are modifying the bare band in a continuous manner but are expected to be weak if graphene is on a metallic substrate because of screening. To extract the bare band for each dopant, we look to the measured spectral functions at an energy that is sufficiently far away from both the electron–phonon and the electron–plasmon renormalizations. This energy was defined as corresponding to the charge transfer of 0.022 electrons per C atom. For example, for Rb, this charge transfer corresponds to a contour 550 meV below the Fermi level, and for the other dopants it is at similar energies. Contours around this energy and the Fermi energy contour have been used to fit the bare band dispersion. To determine the bare band for energies in between, a constrained, self-consistent procedure that yields both the self-energy and the bare band is applied and explained in detail in the next section. Importantly, the choice of the correct bare band is well-defined because, only for one choice of the bare band, the real and imaginary parts of the self-energy, Σ are Kramers-Kronig related. The bare band dispersion obtained in this way contains (i) the effects of the positively charged ions and (ii) the effects of trigonal warping, that is, a different curvature in the KM and Γ K directions. This is important because previous works have shown that a simple, linear bare band causes an apparant anisotropy in the electron–phonon interaction [29] . Let us now investigate whether the bare electron energy band dispersion is identical for all dopants. This experiment is to challenge the applicability of the rigid-band model, which is widely employed for doped carbon materials. This model states that the doping purely results in a Fermi level shift (a bandstructure offset) but no change in the slope of the bands. As we will show below, this is not the case for the present systems. To investigate the applicability of the rigid-band model, we measured surfaces around the K point, which correspond to the same charge transfer of 0.022 electrons per C atom (iso-area contours). Such iso-area surfaces allow us to investigate the dopant-induced changes in the bare band structure independent of electron–phonon and electron–plasmon coupling. If each dopant system would have identical band slopes, the energies (measured from Dirac point) at which the iso-area contours are taken would be equal to each other. As we show below, this is not the case and a marked change in the slope of the bare band dispersion occurs. In Fig. 2b , the aforementioned iso-area contours are shown for each dopant system. Clearly, these contours are not identical and the deviations also follow a clear trend: with increasing doping level, the contours become more trigonally warped. A related effect has been reported previously [24] , [30] , [31] and ascribed to the presence of an electric field of the ionized adatom. In the present case, we ascribe the observed deviations from the rigid-band model to the complex interplay of screening of the dopant ion by graphene and the metallic substrate and the different geometry for each interface where the dopant can be on top of graphene or buried in the graphene–substrate interface (see previous section). The observed changes in the slope of the π bands are important for resonance Raman experiments of doped carbon materials, especially graphene [4] because the resonance process selects certain electron wavevectors according to the photon energy and is therefore sensitive to the band slopes. Electron–phonon coupling It is widely established, that the Eliashberg function α 2 F ( ω , ε, k ), which contains the phonon density of states F ( ω ) and the scattering probability for a photohole [32] , α 2 governs EPC and can be successfully probed by ARPES. The fundamental parameter λ , which describes the strength of EPC, can be estimated according to From the above Equation 1, it is clear that a high λ requires low-energy phonons since these are dominant because the 1/ ω dependence gives larger contributions for smaller ω . In classical Bardeen–Cooper–Schrieffer (BCS) theory, λ is related to the transition temperature T c via the McMillan formula [33] . Hence, the Eliashberg function α 2 F ( ω , ε, k ) contains all we need to predict T c . It has been shown for Be [26] and also for graphene [27] that α 2 F ( ω , ε, k ) can be extracted from high-quality ARPES data. Regarding graphene, we have shown previously [27] that α 2 F ( ω , ε, k ) contains an isotropic contribution in both high-symmetry directions of two peaks for the graphene-derived optical phonons from Γ and K points while an extra low-energy peak appears in KM direction only. On the basis of these results, we modelled the Eliashberg functions in Γ K and KM direction with a sum of two and three Lorentzian lines, respectively. As we will show below, it is this low-energy part in KM direction that is key to achieving high EPC. The first step of the analysis procedure is to extract the real and imaginary part of the self-energy from the momentum dispersion curves (MDCs) using a polynomial bare dispersion according to ref. 34 : and Here k is the peak position of the Lorentzian distribution, Δ k is the half width at half maximum and υ 0 ( ω ) is a bare electron velocity. The choice of the bare band is crucial and plays a significant role in determining the lineshape and magnitude of the self-energy. We therefore used a self-consistent way in which we calculate the Eliashberg function as the sum of Lorentzian functions for each choice of the bare band and model the self-energy from it. The bare band that yields the smallest deviation in the calculated self-energy is then employed. The imaginary part of the self-energy and the Eliashberg function are related via [32] Here, f and n are the Fermi and Bose distribution functions, respectively. Therefore the determination of α 2 F ( ω , ε, k ) requires an integral inversion, which we have performed numerically with the constraints that α 2 F ( ω , ε, k ) can be expressed as a sum of Lorentzians and that the bare band has negative curvature in KM direction and positive curvature in Γ K direction. Using the numerical integral inversion, we can extract α 2 F ( ω , ε, k ). It is considered successful if the ℑ Σ and ℜ Σ calculated from the extracted α 2 F ( ω ,ε, k ) match the experimental one. The high-resolution ARPES measurements in the kink region in the Γ K and KM high-symmetry directions are shown in Fig. 2c . These highly resolved data allow for an extraction of Σ by the method outlined above. The fully Kramers–Kronig consistent ℜ Σ and ℑ Σ are displayed in Fig. 3 along with the Eliashberg function. The dopant-dependent Eliashberg functions are the core result of our work and key to understanding EPC and superconductivity in doped graphene. A set of two (three) Lorentzians with a half-width at half-maximum of 11±1 meV is sufficient to model Σ in excellent agreement to the experiment in the Γ K ( KM ) direction. The extra low-energy peak in KM is seen best for Ca as a shoulder in ℜ Σ and an additional step in ℑ Σ. 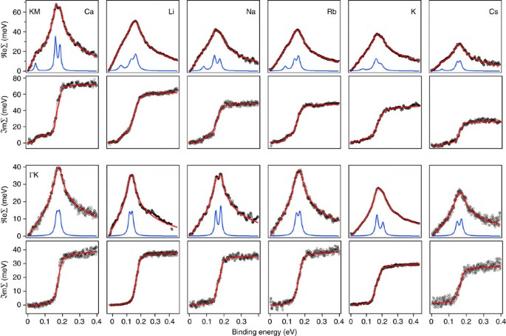Figure 3: Analysis of electron–phonon coupling. The complex self-energy Σ along with the Eliashberg function forKMand ΓKdirections. Black dots denote the experimental data and red lines the calculated Σ. The blue line below the real part of Σ is the Eliashberg function. Figure 3: Analysis of electron–phonon coupling. The complex self-energy Σ along with the Eliashberg function for KM and Γ K directions. Black dots denote the experimental data and red lines the calculated Σ. The blue line below the real part of Σ is the Eliashberg function. Full size image All Eliashberg functions in KM direction are plotted in Fig. 4a , highlighting the strong individuality of the low-energy peak, which remarkably depends on the dopant. The high-energy peaks for all alkalis are practically at the same energy, except for Ca. The increase of the high-energy phonons of Ca-doped graphene is most probably due to the more significant weakening of the Kohn anomaly with doping which causes an upshift in the phonon energy [35] . The strong and inhomogeneous dopant dependence of the low-energy peak in the Eliashberg function points towards dopant-derived phonons and will be analyzed in detail below. Let us first focus on the dopant dependence of λ shown in Fig. 4b,c for Γ K and KM directions, respectively. It can be seen that (i) the value of λ increases with the doping level and is largest for Ca and (ii) there is a marked asymmetry in KM and Γ K directions, which is also largest for Ca. From the linear energy dependence of the density of states in graphene, one can expect a square root behaviour of EPC with increasing of the charge carrier population [36] . It is clear from Fig. 4b that the Γ K direction follows this behaviour with small deviations that are probably related to the peculiarities of each dopant. However, for the KM direction shown in Fig. 4c , this model completely fails and λ rises much faster with carrier concentration than the expected square root law. By integrating the Eliashberg function in KM only over the graphene-derived optical high-energy (HE) phonons, we highlight their contribution to λ as shown in Fig. 4d , which also follows the square root law. From these results it is clear that the EPC constant that comes from graphene’s HE phonons alone is too low to sustain superconductivity, even for Ca-doped graphene. 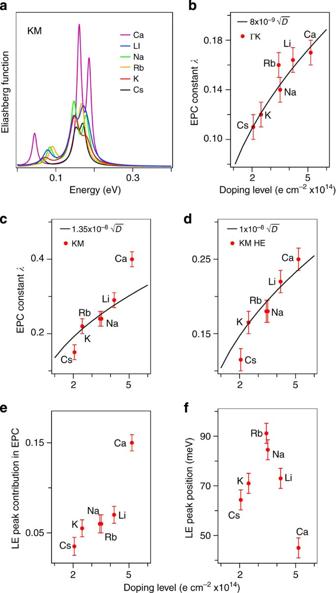Figure 4: Dopant dependence of electron–phonon coupling. (a) ARPES derived Eliashberg functions along theKMdirection for all dopants. (b,c) The dependence of the total EPC on the electron concentration for wave vectors along the ΓKandKMdirections. (d) The contribution of graphene high-energy (HE) optical phonon modes only to EPC inKMdirection. The black line is a fit of the experimental data points to a square root law. (e) Contribution of the low energy (LE) peak in Eliashberg function to the EPC constant. (f) Position of the low energy (LE) peak in Eliashberg function versus doping level. The error bars ofλin (b–e) and the position of the LE feature were estimated from the error in Σ and from the error in the Fermi level position and the energy resolution. Figure 4: Dopant dependence of electron–phonon coupling. ( a ) ARPES derived Eliashberg functions along the KM direction for all dopants. ( b , c ) The dependence of the total EPC on the electron concentration for wave vectors along the Γ K and KM directions. ( d ) The contribution of graphene high-energy (HE) optical phonon modes only to EPC in KM direction. The black line is a fit of the experimental data points to a square root law. ( e ) Contribution of the low energy (LE) peak in Eliashberg function to the EPC constant. ( f ) Position of the low energy (LE) peak in Eliashberg function versus doping level. The error bars of λ in ( b – e ) and the position of the LE feature were estimated from the error in Σ and from the error in the Fermi level position and the energy resolution. Full size image This raises important questions regarding the origin of the low-energy phonon in KM direction, which we are able to answer conclusively in this work. Two scenarios are conceivable: (i) a graphene-related acoustic phonon which can fulfill energy-momentum conservation rules for intravalley scattering and (ii) a dopant atom related vibration. Here we bring forward compelling reasons that dismiss case (i) and point towards the scenario with a dopant atom induced phonon. If scenario (i) were the case, the dopant-dependent contribution to EPC of the low-energy peak must follow the square root law as it was the case for the graphene-related optical phonons shown in Fig. 4b and in Fig. 4d . However, as we show in Fig. 4e , the contribution to EPC of the low-energy phonon is substantially different from a square root law. Moreover, if scenario (i) would be the case, energy-momentum conservation dictates that the position of the low-energy phonon would follow the slope of the acoustic phonon branches in graphene. This would invariably lead to an increase of the position of the low-energy peak with increasing doping level because larger phonon wave vectors (and hence energies) are required to couple states on a larger Fermi surface. However, in our experiment the opposite is the case as we show in Fig. 4f . It is clear that the energy of the low-energy feature first rises with doping but then changes slope and decreases after a doping level of ∼ 3 × 10 14 e cm −2 yielding the lowest energy in Ca-doped graphene. Interestingly, the position of the low-energy feature does not follow a simple trend. This might be expected from the frequency of a simple oscillator model that is equal to with a dopant-independent force constant k between graphene and the ion with mass m . However, k might depend in a complex manner on (1) degree of ionization, the (2) distance of the ion to graphene and (3) whether the ion is on top or under graphene. Therefore, we think that this is the reason why no easy relation between the dopant mass and the frequency can be observed. We now move to the implications of the extracted λ on superconductivity. On the basis of the values of λ in KM direction, estimations of the superconducting transition temperature T c were calculated according to the McMillan formula with a screened Coulomb pseudopotential μ *=0.14 (ref. 19 ; see Methods section). Table 1 lists the results for all dopants used in this study. We found that Ca-doped graphene has the largest value T c =1.5 K and from our preceding analysis it is clear that the high EPC is dominated by the low-energetic peak that is present for all dopants but strongest for Ca. Apparently, it is not a matter of the Fermi surface size alone: the Li-doped graphene has a similar value of carrier density but a substantially smaller λ . We therefore assume that modifications of the graphene-substrate interface by Ca provide a change of the local potential that causes the observed changes in the Eliashberg function. Table 1 Summarized results obtained from ARPES measurements of doped graphene. Full size table Let us discuss our results in the light of superconductivity in GICs, which is also induced by EPC. First, the ARPES measurements of EPC in GICs yield much higher values than for the doped graphene with a similar stoichiometry. For example, in KC 8 the values of λ range from λ =0.33 to λ =0.91, with the momentum-averaged value of λ =0.45 (ref. 37 ). This is considerably higher than present case of the K-doped monolayer. A similar situation is the case for the Ca dopant, for which also ARPES data exist. In the case of bulk CaC 6 , the values of λ range from 0.38 to 0.89, with the momentum-averaged value of 0.53 (ref. 34 ). Again, this is considerably higher than the monolayer case. We ascribe this difference to the three dimensional nature of the GIC compound and more specifically to three reasons. First, the intercalation of dopant atoms in between graphene sheets enhances the dopant order. This is evident for the case of Ca. For example, Ca is disordered on monolayer graphene on SiC (ref. 24 ) and in the present case while it is ordered in GICs and in intercalated few-layer graphene [25] (evidenced by diffraction measurements). This in turn might enhance formation of interlayer bands, which will increase λ by providing the additional electronic states for scattering. Second, the existence of more than one layer provides additional phonon modes for the coupling (graphene layers vibrating against each other), which have a sizable coupling to the interlayer state [23] and can also increase λ . Third, in the case of the CaC 6 bulk compound, the doping level is slightly higher than in the present case, which in turn can lead to nesting, further increasing λ (ref. 34 ). Let us focus now on calculations of EPC and the prediction of superconductivity in alkali metal-doped monolayer graphene by Profeta et al. [22] EPC in the systems we have studied depends in a complex way on various factors [22] : distance of the dopants from the graphene layer and confinement of the dopant wave function, which both determine the position of the interlayer band relative to the Fermi level; the phonon frequency and mass of the dopant ions; the density of states at the Fermi level, which is determined by the charge carrier concentration. In addition, there are crucial differences between the theoretically and experimentally treated system and therefore the comparision with the calculations must be done with caution. First, in the experiment, the graphene is on a substrate while it is freestanding in the calculation. This difference can modify the shape of the interlayer state wavefunction, which in turn has a large influence on λ . Notably, it is the absence of a confining potential in the case of Li-doped graphene that causes the large values of calculated T c (ref. 22 ). Second, the dopant adsorbates are perfectly ordered in the calculation, while this is not the case in our experiments. Moreover, in some systems (K and Ca) the dopants are below the graphene sheet and in direct contact to the metallic substrate that can act as an electron acceptor. The possibility of ionization from the Au substrate and the disorder have strong effects on the interlayer state and can even cause it to disappear. This is one mechanism by which the experimental λ would become smaller than the theoretical value. A comparison of the theoretical and experimental values of λ for Ca yields a very good agreement in KM direction (expt. λ KM =0.4, λ ΓK =0.17, theory λ =0.4). Regarding Li, the discrepancies are more obvious (expt. λ KM =0.29, λ ΓK =0.16, theory λ =0.61) and they are ascribed to the reasons stated above. The obtained results have a palpable impact on achieving superconductivity in 2D materials in general and for functionalized graphene systems in particular. Regarding the outlook of this research direction and future experiments using different methods, it would be interesting to study the effect of large doping levels without the presence of dopant ions. Such an experiment would provide additional proof of the role of dopant vibrations. These experiments could be done using field effect gating or organic electrolytes in an electric double-layer system [38] . Photoemission measurements The XPS measurements were carried out at the German-Russian beamline (RGBL) of the BESSY II synchrotron in Berlin (Germany) collecting electrons in normal emission and with an emission angle of 60° with respect to the sample surface. ARPES measurements of samples prepared in an identical manner were carried out at the BaDElPh beamline [39] of the Elettra synchrotron in Trieste (Italy). ARPES spectra were acquired at a photon energy of 29 eV with the sample held at 50 K and a base pressure better than 5 × 10 −11 mbar. The total angular and energy resolution was determined to 0.15° and 15 meV, respectively. Because of matrix element effects in the photoemission cross section, the π* graphene states are invisible with p polarization in the first Brillouin zone. Hence, we performed our photoemission studies in both, p and s polarization. Sample preparation Pristine graphene samples were prepared in situ under ultra high vacuum conditions with chemical vapour deposition of propylene on Ni(111) thin films on W(110) single crystals followed by intercalation of one monolayer (ML) Au [7] , [40] , [41] . We evaporated alkali metals from commercial SAES getters and Ca from a Ta crucible onto graphene followed by annealing. The dopant concentration was increased stepwise and after each dopant evaporation the downshift in the C 1 s core level was recorded using XPS. Only after the C 1 s line position was not shifting any more upon increasing the dopant concentration, we considered the sample to be fully doped. The total amount deposited corresponded to ∼ 1 Ml in the case of alkali metals and ∼ 3 Ml for Ca according to quartz microbalance and XPS. The two observed values were in agreement within an error of 15%. The crystal quality was checked by low-energy electron diffraction (LEED) for each step in the synthesis procedure. We found a sharp LEED pattern for W(110), Ni(111)/W(110), graphene/Ni(111)/W(110) and graphene/Au/Ni(111)/W(110) but no LEED pattern corresponding to the dopants. Data analysis The stoichiometry was determined using XPS in the framework of a two layer system (graphene/dopant). Via rotational and mirror symmetry operations with respect to the K point we could cross-check several reconstructed Fermi surfaces and perform a fit to the photoemission maxima. To estimate the position of Dirac point, we performed momentum distribution curve (MDC) analysis with Lorentzian functions for both polarization ARPES spectra separately and added them together at the same plot. Estimation of the superconducting transition temperature In classical Bardeen–Cooper–Schrieffer (BCS) theory, λ is related to the transition temperature T c via the McMillan formula Here the approximation on the right side is valid for small λ with μ * being the screened pseudopotential and ‹Θ› the average phonon temperature that is given by where k B is the Boltzmann constant. On the basis of the experimentally extracted Eliashberg functions, we performed estimations of the T c values that are summarized in the Table 1 . How to cite this article: Fedorov, A. V. et al. Observation of a universal donor-dependent vibrational mode in graphene. Nat. Commun. 5:3257 doi: 10.1038/ncomms4257 (2014).